Pore-opening mechanism in trimeric P2X receptor channels The opening of ion channels in response to ligand binding, voltage or membrane stretch underlies electrical and chemical signalling throughout biology. Two structural classes of pore-opening mechanisms have been established, including bending of pore-lining helices in the case of tetrameric cation channels, or tilting of such helices in mechanosensitive channels. In this paper, we explore how the structure of the pore changes during opening in P2X receptors by measuring the modification of introduced cysteine residues in transmembrane helices by thiol-reactive reagents, and by engineering metal bridges. Our results are consistent with the X-ray structure of the closed state, and demonstrate that expansion of the gate region in the external pore is accompanied by a significant narrowing of the inner pore, indicating that pore-forming helices straighten on ATP binding to open the channel. This unique pore-opening mechanism has fundamental implications for the role of subunit interfaces in the gating mechanism of P2X receptors and points to a role of the internal pore in ion permeation. Ion channels are membrane proteins that contain ion-selective pores through which sodium, potassium, calcium or chloride ions can enter or exit the cell through diffusion. The pore in most ion channels opens and closes in response to specific stimuli, such as the binding of a ligand, changes in membrane voltage or stretching of the membrane. In tetrameric cation channels, including several types of potassium channels [1] , [2] , [3] , [4] , [5] , [6] , and the NaK channel from Bacillus cereus [7] , the outer end of the pore containing the selectivity filter remains relatively stationary (but moves during a process termed inactivation [3] , [8] ), whereas the internal pore-lining helices bend outwards and rotate to open the pore. In mechanosensitive channels [9] , [10] , [11] , [12] , [13] , [14] pore-lining helices tilt towards the plane of the bilayer as they are pulled laterally to open the pore. In contrast, very little is known about the opening mechanism in trimeric cation channels, such as P2X receptor channels, acid-sensing ion channels or epithelial sodium channel, although several recent X-ray structures for these distantly related proteins provide a new framework for exploring their pore-opening mechanisms [15] , [16] , [17] . The X-ray crystal structure of an ATP-activated P2X receptor channel from zebrafish (zfP2X4) reveals that the ligand-free protein is comprised of a transmembrane domain containing two transmembrane (TM) helices per subunit, and a extracellular domain housing three ATP-binding sites [15] . Each subunit adopts a porpoise-like structure that wraps around one another in the trimeric complex ( Fig. 1a ). The pore-lining TM2 helices [18] , [19] , [20] , [21] , [22] , [23] , [24] , [25] , [26] , [27] , [28] , [29] are arranged around the three-fold axis of molecular symmetry and are unusual in that they are steeply angled (~50 degrees) relative to the normal of the membrane plane ( Fig. 1a,b ), a feature that distinguishes this closed-state structure from those of tetrameric and pentameric ion channels [7] , [9] , [30] , [31] . These TM2 helices cross in the outer half of the membrane, giving the pore an hourglass appearance, with a constriction formed by three residues in the TM2 helix (L340, A344 and A347 in zfP2X4), flanked by solvent-accessible vestibules near the external and internal surfaces ( Fig. 1b ). The presence of occlusion in the outer pore of the zfP2X4 channel is consistent with functional studies examining the location of the gate region within TM2 of the rat P2X2 (rP2X2) receptor channel [28] , [32] indicating that the occlusion observed in the structure actually functions as a gate to control entry of ions into the pore. The aim of this study was to understand how the structure of the pore changes in response to ATP binding to the extracellular domain. We began by exploring the extent of structural changes in the pore by studying the solvent accessibility of cysteine (Cys) residues introduced throughout TM1 and TM2. We also estimated the extent to which the gate region expands by studying accessibility in this region to large thiol-reactive compounds. Finally, we explored whether metal bridges could be formed between introduced Cys residues in the pore-lining TM2 helix and determined the coordinating side chains for two Cd 2+ bridges formed within the internal pore region. Our results lead us to propose a new type of pore-opening model in which TM2 helices straighten to enlarge the outer pore while constricting the inner pore. 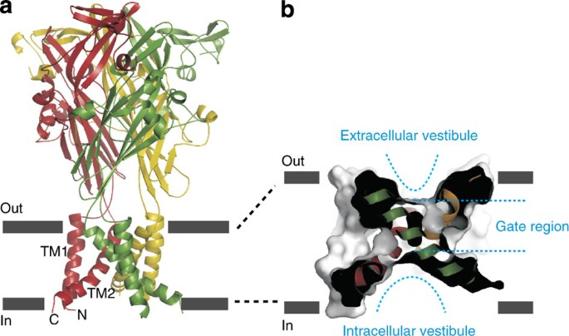Figure 1: The architecture of the P2X receptor channel and the pore domain. (a) Backbone structure of the zfP2X4 receptor viewed parallel to the membrane showing that these proteins are trimers with a large extracellular domain and a relatively small transmembrane domain in each subunit. (b) A sagittal section of a surface rendering of the transmembrane domain shows that the closed pore formed by angled TM2 helices has an hourglass shape, with vestibules on each side of a gate located within the external half of the membrane. All structures in this and subsequent figures were drawn using PDB accession code3H9Vand PyMol (DeLano Scientific.). Figure 1: The architecture of the P2X receptor channel and the pore domain. ( a ) Backbone structure of the zfP2X4 receptor viewed parallel to the membrane showing that these proteins are trimers with a large extracellular domain and a relatively small transmembrane domain in each subunit. ( b ) A sagittal section of a surface rendering of the transmembrane domain shows that the closed pore formed by angled TM2 helices has an hourglass shape, with vestibules on each side of a gate located within the external half of the membrane. All structures in this and subsequent figures were drawn using PDB accession code 3H9V and PyMol (DeLano Scientific.). Full size image Silver modification rates in closed and open states In a previous accessibility study of the two TMs of rP2X2 receptor channels [28] , we explored the modification of introduced Cys residues to the thiol-reactive compound 2-trimethylaminoethyl methanethiosulphonate (MTSET) applied to the external side of the channel, and identified one reactive position in TM1 and seven in TM2. Further measurements of the rates of modification of the seven positions in TM2 with external Ag + ions [28] , a small thiol-reactive ion that rapidly and covalently modifies water-exposed Cys residues [33] , [34] demonstrated that these residues are rapidly modified in the open state (4.8×10 7 to 5.2×10 8 M −1 s −1 ), suggesting that they line the ion permeation pathway. Comparison of the rates of modification in both the absence and presence of ATP suggested that an extended gate is located between I332 and I341 ( Fig. 2b ; grey symbols), consistent with the structure of the zfP2X4 receptor. Our initial objective in this study was to determine the extent to which the structure of the pore changes during opening. Is the structural change highly localized or are there widespread rearrangements within the pore? 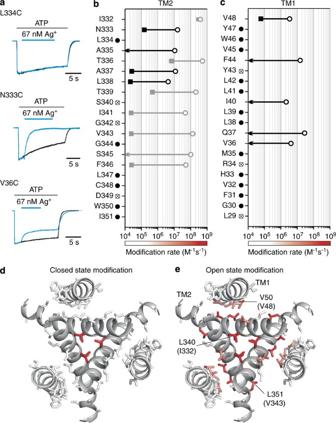Figure 2: State-dependent accessibility of extracellular Ag+in rP2X2 receptor channels. (a) Examples showing distinct effects of extracellular Ag+for channels with Cys substitutions at three different positions. In the presence of saturating concentrations of ATP28, L334C was insensitive to Ag+, whereas N333C and V36C currents were inhibited when Ag+is applied. Black current traces are controls recorded by applying ATP alone. Blue current traces were recorded 2 min after the control, and Ag+was applied as indicated by the blue bars. Currents were scaled and superimposed to show the effects of Ag+. (b) and (c) Ag+modification rates for Cys substitutions throughout TM1 and TM2. Data from Liet al.28are shown as grey symbols for comparison. Open circles represent modification rates obtained in the presence of saturating concentrations of ATP (0.3–30 μM) and filled squares represent modification rates obtained in the absence of ATP (n=4–6; error bars are s.e.m. and are smaller than the symbols). Arrows indicate that there is no observable effect, when 67 nM Ag+was applied for 2 min in the absence of ATP. Filled black circles indicate that 67 nM Ag+has no detectable effect on the Cys substitution either in the presence or in the absence of ATP. Cys mutations with crossed circles either give little response to 100 μM ATP or desensitize very fast. (d) and (e) Mapping of Ag+modification rates onto transmembrane helices in the zfP2X4 structure (viewed from the extracellular side) reveals the dramatic change in solvent accessibility when channel opens. Residues are coloured using a continuous colour gradient from white to red to represent Ag+modification rates, as indicated by the coloured bars shown at the bottom of (b) and (c). V50, L340 and L351 are labelled on the zfP2X4 structure, which correspond to V48, I332 and V343 in rP2X2. Figure 2: State-dependent accessibility of extracellular Ag + in rP2X2 receptor channels. ( a ) Examples showing distinct effects of extracellular Ag + for channels with Cys substitutions at three different positions. In the presence of saturating concentrations of ATP [28] , L334C was insensitive to Ag + , whereas N333C and V36C currents were inhibited when Ag + is applied. Black current traces are controls recorded by applying ATP alone. Blue current traces were recorded 2 min after the control, and Ag + was applied as indicated by the blue bars. Currents were scaled and superimposed to show the effects of Ag + . ( b ) and ( c ) Ag + modification rates for Cys substitutions throughout TM1 and TM2. Data from Li et al . [28] are shown as grey symbols for comparison. Open circles represent modification rates obtained in the presence of saturating concentrations of ATP (0.3–30 μM) and filled squares represent modification rates obtained in the absence of ATP ( n =4–6; error bars are s.e.m. and are smaller than the symbols). Arrows indicate that there is no observable effect, when 67 nM Ag + was applied for 2 min in the absence of ATP. Filled black circles indicate that 67 nM Ag + has no detectable effect on the Cys substitution either in the presence or in the absence of ATP. Cys mutations with crossed circles either give little response to 100 μM ATP or desensitize very fast. ( d ) and ( e ) Mapping of Ag + modification rates onto transmembrane helices in the zfP2X4 structure (viewed from the extracellular side) reveals the dramatic change in solvent accessibility when channel opens. Residues are coloured using a continuous colour gradient from white to red to represent Ag + modification rates, as indicated by the coloured bars shown at the bottom of ( b ) and ( c ). V50, L340 and L351 are labelled on the zfP2X4 structure, which correspond to V48, I332 and V343 in rP2X2. Full size image To address these questions, we measured the rates of external Ag + modification for Cys residues introduced at each position in TM1 and TM2. Although our earlier experiments with MTSET as a reactive probe identified relatively few reactive positions [28] , Ag + is much smaller and therefore improves the effective resolution with which we can probe for structural changes. In TM1, we identified five positions at which Ag + modified channels in the presence of ATP (2.1×10 6 to 2.8×10 7 M −1 s −1 ), and in each instance, modification in the absence of ATP was either slow or could not be observed (modification rate <10 4 M −1 s −1 ; Fig. 2c , black arrows). For the remaining 15 positions, 12 displayed no measurable modification by Ag + in either open or closed states (filled circles), and three mutants could not be studied because ATP-activated currents were too small to be studied (crossed circles). In TM2, we identified four additional positions at which Ag + modified channels in the presence of ATP (4.2×10 6 to 1.6×10 7 M −1 s −1 ), and in each case, the modification rate was dramatically slower in the absence of ATP ( Fig. 2b , black filled squares or arrows). There were only six positions in TM2 at which Ag + modification could not be detected, and three that could not be studied, either because the mutants did not display ATP-activated currents or they rapidly desensitized, a process by which channels enter a non-conducting state in the continual presence of ATP [35] . If we map the collective Ag + modification rates for the closed and open states onto the structure of the closed zfP2X4 receptor channel using a continuous colour gradient from white (≤10 5 M −1 s −1 ) to red (10 9 M −1 s −1 ), several informative patterns emerge. First, the vast majority of residues in TM1 and TM2 exhibit slow (10 4 –10 5 M −1 s −1 ) or undetectable modification by Ag + in the absence of ATP ( Fig. 2d ), which is consistent with the X-ray structure in which most of these residues have limited solvent exposure because they are buried in the protein or line the internal vestibule below the gate. The very rapid modification observed for I332C in the absence of ATP is consistent with the crystal structure in which the equivalent residue (L340 in zfP2X4) forms the outer edge of the occlusion and is solvent exposed. In the case of T336C, the relatively rapid modification we observed in the absence of ATP can be explained by the spontaneous opening observed in this mutant [29] . Second, there is a general increase in modification rate on opening for TM2 residues involved in packing in the external region between I332 and T339, indicating that the entire external region of TM2 becomes more solvent accessible when the channel opens ( Fig. 2d,e ). Residues that line the external pore in the closed state structure also exhibit the most rapid Ag + modification rates in the open state, indicating that any rotation of the TM2 helix during opening [26] , [29] must be less than one α -helical turn (100°). Third, although most residues in TM1 do not exhibit measurable Ag + accessibility in either closed or open states, the five accessible positions exhibit moderate modification rates (10 6 –10 7 M −1 s −1 ) and map to a single face of the TM1 helix. The Ag + accessible face of TM1 is interesting because it packs with the backside of TM2 in the closed state structure, and therefore would not be expected to exhibit significant Ag + accessibility unless the spatial relationship between TM1 and TM2 changes as the pore opens (see Discussion ). Viewed collectively, the Ag + modification results suggest that the structure of the pore in P2X receptor channels undergoes widespread rearrangements during opening. Gauging expansion of the gate region during opening To determine the extent to which the external pore expands within the gate region of TM2 when the channel opens, we tested for modification of T336C and T339C by two large methanethiosulphonate (MTS) reagents, 2-tripentylaminoethyl MTS (MTS-TPAE) and Texas Red-MTSEA (TR-MTSEA) [34] ( Fig. 3a ). In the presence of ATP, both residues can be modified by MTS-TPAE with rates (2.5 ± 0.03×10 4 for T336C, n =4; 1.4 ± 0.15×10 4 M −1 s −1 for T339C, n =4) similar to those observed for smaller MTS reagents [28] ( Fig. 3b,c ). Although T336C can be modified by TR-MTSEA, a larger mushroom-shaped reagent with a relatively rigid pileus and a sulphydryl-reactive group at the base of the stem, modification of T339C could not be observed. These results suggest that the diameter of the gate region of the pore in the open state is somewhat smaller than the dimensions of the pileus of TR-MTSEA (~13 Å). 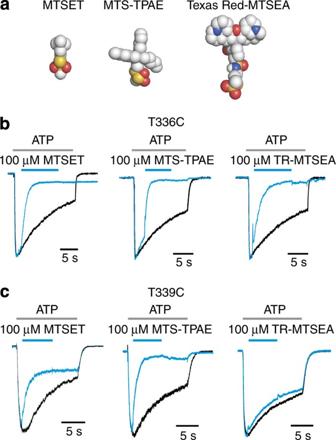Figure 3: Modification of T336C and T339C by MTS reagents of various sizes. (a) Molecular models for the reagents tested with carbon-coloured grey, oxygen red, nitrogen blue and sulphur yellow. (b) Superimposed scaled current traces demonstrate that T336C can be modified by all three MTS reagents shown in (a). Black current trace was recorded first by applying ATP alone, and blue current trace was recorded 2 min later by applying MTS reagents in the presence of ATP, as indicated by the bars above the current traces. (c) Superimposed scaled current traces show that T339C can be modified by MTSET and MTS-TPAE, but not by TR-MTSEA. EC50concentrations of ATP28were used in each experiment (9 μM for T336C and 3 μM for T339C), and similar results were obtained in 4–12 different experiments. Figure 3: Modification of T336C and T339C by MTS reagents of various sizes. ( a ) Molecular models for the reagents tested with carbon-coloured grey, oxygen red, nitrogen blue and sulphur yellow. ( b ) Superimposed scaled current traces demonstrate that T336C can be modified by all three MTS reagents shown in ( a ). Black current trace was recorded first by applying ATP alone, and blue current trace was recorded 2 min later by applying MTS reagents in the presence of ATP, as indicated by the bars above the current traces. ( c ) Superimposed scaled current traces show that T339C can be modified by MTSET and MTS-TPAE, but not by TR-MTSEA. EC 50 concentrations of ATP [28] were used in each experiment (9 μM for T336C and 3 μM for T339C), and similar results were obtained in 4–12 different experiments. Full size image Engineering cadmium bridges with pore-lining residues To explore the manner in which the pore-lining TM2 helix moves during opening, we asked whether non-covalent Cd 2+ bridges could be formed between introduced Cys residues. In studies on the tetrameric Shaker Kv channel [34] , [36] , Cd 2+ can be stably coordinated by three or four Cys residues at the central axis of the pore when Cys is introduced at a single position within the pore-lining helix of all four subunits. We began by studying residues in the outer gate region of TM2 (I332C, T336C and T339C) because they are positioned close to the central axis in the closed state and can be rapidly modified by Ag + in the open state ( Fig. 2b,d,e ). For these three positions, we observed inhibition of the channel for short (300 ms) applications of Cd 2+ to the extracellular solution in the presence of ATP; however, in each case, the channel recovered rapidly on removing the metal, indicating that coordination was relatively weak ( Supplementary Fig. S1 ). For T336C, longer applications of Cd 2+ (1 or 8 s) caused a fraction of channels to recover slowly, as previously reported [28] , which may result from stable coordination of Cd 2+ in the desensitized state ( Supplementary Fig. S1 ). For I332C and T339C, recovery remained rapid after longer applications of Cd 2+ , but channels recovered to a larger extent than would be expected from the amount of desensitization seen in control solutions ( Supplementary Fig. S1 ), as if weak Cd 2+ coordination at these positions prevents desensitization. Although the effects of Cd 2+ at these three positions suggest that the gate region within TM2 moves during desensitization, they do not provide reliable constraints for the open state of the channel because the unstable coordination we see following brief applications of Cd 2+ could result from metal coordination by only one or two Cys residues. We also tested for Cd 2+ coordination by Cys at other positions within the external region of TM2 that displayed measurable Ag + accessibility (I328C, N333C, A335C, A337C and L338C; Supplementary Fig. S2 ); however, in each case, application of Cd 2+ had no detectable effect. Having failed to uncover positions at which Cys residues could stably coordinate Cd 2+ in the open state within the external region of TM2, we turned our attention to the internal pore. Although Ag + also rapidly modifies Cys residues substituted at three positions within the internal region of TM2 (V343C, S345C and F346C; Fig. 2b ), these residues are too far apart (Cβ–Cβ distances of 18 to 23 Å) in the closed state structure to coordinate Cd 2+ ( Fig. 4e ). Remarkably, however, external application of Cd 2+ in the presence of ATP caused a robust inhibition of channels with Cys substitutions at V343, and the channel recovered slowly after removal of the metal ( Fig. 4a ; Supplementary Fig. S3 ), even after brief applications of Cd 2+ ( Supplementary Fig. S1e ). The association rate for Cd 2+ inhibition at this position is rapid (1.6±0.01×10 6 M −1 s −1 , n =6; Fig. 4d ), somewhat faster than observed within the intracellular gate region of open Shaker Kv channels [34] , suggesting that stable coordination takes place in the open state of P2X receptor channels. Stable coordination of Cd 2+ was also observed at S345 and F346 ( Fig. 4b,c,d ), although the association rates and apparent affinities at these positions are much lower than for V343C, leaving the state in which the bridges form undefined. 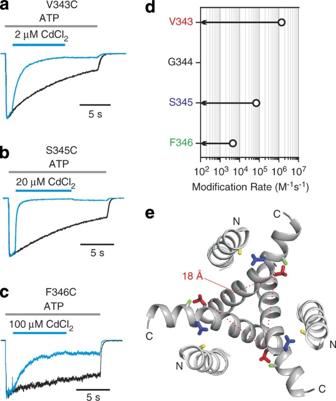Figure 4: Stable Cd2+coordination at V343, S345 and F346. (a) Superimposed scaled current traces show that V343C current is rapidly inhibited by 2 μM CdCl2, and the inhibition recovers slowly after removal of Cd2+. (b) and (c) Superimposed scaled current traces show that S345C and F346C currents are inhibited by applying 20 or 100 μM CdCl2, and the inhibition is only slowly reversible. (d) Summary of stable Cd2+coordination rates. Open circles represent the stable coordination rates of Cd2+in the presence of ATP (n=4–6; error bars are s.e.m. and are smaller than the symbols). Arrows indicate that there is no detectable effect of 20 μM CdCl2on ATP-activated currents when applied for 2 min in the absence of ATP. In all cases, saturating concentrations of ATP28were used to activate the channel (30 μM for V343C containing channels and 100 μM for S345C and F346C). (e) TM helices viewed from the intracellular side of the membrane. V343, S345, F346 and H33 are labelled in red, blue, green and yellow, respectively. The Cβ–Cβ distance of V343 from three subunits is indicated by dotted lines. Figure 4: Stable Cd 2+ coordination at V343, S345 and F346. ( a ) Superimposed scaled current traces show that V343C current is rapidly inhibited by 2 μM CdCl 2 , and the inhibition recovers slowly after removal of Cd 2+ . ( b ) and ( c ) Superimposed scaled current traces show that S345C and F346C currents are inhibited by applying 20 or 100 μM CdCl 2 , and the inhibition is only slowly reversible. ( d ) Summary of stable Cd 2+ coordination rates. Open circles represent the stable coordination rates of Cd 2+ in the presence of ATP ( n =4–6; error bars are s.e.m. and are smaller than the symbols). Arrows indicate that there is no detectable effect of 20 μM CdCl 2 on ATP-activated currents when applied for 2 min in the absence of ATP. In all cases, saturating concentrations of ATP [28] were used to activate the channel (30 μM for V343C containing channels and 100 μM for S345C and F346C). ( e ) TM helices viewed from the intracellular side of the membrane. V343, S345, F346 and H33 are labelled in red, blue, green and yellow, respectively. The Cβ–Cβ distance of V343 from three subunits is indicated by dotted lines. Full size image Determination of coordinating residues for metal bridges One possible interpretation of the stable bridges formed when Cys is introduced into TM2 is that three Cys residues form a Cd 2+ coordination site at the central axis of the pore. An alternate possibility is that coordination occurs off the central axis, perhaps involving other coordinating atoms that are already present in the background construct in which Cys residues are introduced. Although we removed the one native Cys in TM2 (C348T) in the construct used in our experiments, a His residue (H33) is present within the internal region of TM1, and the zfP2X4 structure would predict that it is positioned near the positions in TM2 at which Cys substitutions result in stable Cd 2+ coordination ( Fig. 4e ). His residues commonly contribute to metal bridges with Cys residues [37] , and its role therefore requires investigation. To test whether three Cys residues are required for stable coordination at V343C, we examined the effects of Cd 2+ on concatamers containing three copies of the rP2X2 sequence, but with different combinations of subunits with and without the V343C mutation. At a concentration that nearly completely inhibits channels containing three V343C subunits (expressed as a single subunit or as a trimeric concatamer), Cd 2+ has little if any effect on channels containing one (1C+2 V) or two (2C+1 V) mutant subunits ( Fig. 5a ; Supplementary Fig. S4 ), demonstrating that three Cys residues are required for stable coordination at this position. For V343C, mutating H33 in TM1 to Tyr did not disrupt stable coordination by Cd 2+ , although we observed a modest twofold slowing of the rate of bridge formation ( Fig. 5b ) that could be explained by an effect of the His mutant on open probability of the channel. We also investigated the number of Cys residues required for stable coordination in S345C; however, in this instance, we observed that stable coordination could still be observed with only two Cys residues. In the case of S345C, mutation of H33 completely disrupts stable coordination even when all three subunits harbour Cys, demonstrating that, in this case, the Cd 2+ bridge is not formed by three Cys residues at the central axis of the pore. 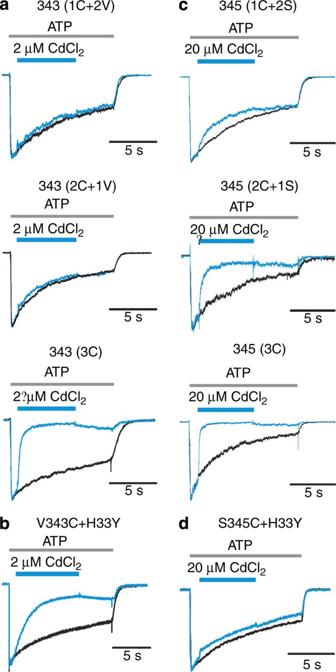Figure 5: Determination of coordinating residues for metal bridges at V343 and S345. (a) Superimposed scaled current traces demonstrate that three Cys are needed at position V343 for stable Cd2+coordination. The concatamer with Cys mutations at V343 in only one or two of the three subunits is not sensitive to 2 μM of CdCl2. (b) Superimposed scaled current traces demonstrate that H33 is not required for tight Cd2+bridge formation at residue V343. (c) Superimposed scaled current traces show that two Cys are sufficient for stable Cd2+coordination at residue S345. (d) Superimposed scaled current traces demonstrate that H33 is involved in tight Cd2+coordination at residue S345. Figure 5: Determination of coordinating residues for metal bridges at V343 and S345. ( a ) Superimposed scaled current traces demonstrate that three Cys are needed at position V343 for stable Cd 2+ coordination. The concatamer with Cys mutations at V343 in only one or two of the three subunits is not sensitive to 2 μM of CdCl 2 . ( b ) Superimposed scaled current traces demonstrate that H33 is not required for tight Cd 2+ bridge formation at residue V343. ( c ) Superimposed scaled current traces show that two Cys are sufficient for stable Cd 2+ coordination at residue S345. ( d ) Superimposed scaled current traces demonstrate that H33 is involved in tight Cd 2+ coordination at residue S345. Full size image The present accessibility and metal-bridging results provide several important structural constraints for the pore of P2X receptor channels. The collective Ag + accessibility results obtained in the absence of ATP are fully consistent with the crystal structure of the zfP2X4 receptors, and the changes observed in the presence of ATP demonstrate that there are widespread rearrangements of TM helices during opening. The residues in TM2 that display the most rapid Ag + modification rates in the open state are also positioned at the central axis of the pore in the closed state structure, indicating that the TM2 helix does not undergo large rotations during opening. One of the unexpected features of these changes in Ag + accessibility is that the face of TM1 that packs with TM2 becomes accessible to Ag + in the presence of ATP, demonstrating that the structural relationship between these helices must change when the channel opens. Our results with MTS-TPAE and TR-MTSEA reveal that the gate region of TM2 expands sufficiently to allow MTS-TPAE to rapidly react with T339C, the deepest residues in the occluded region of the zfP2X4 structure. Finally, the rapid (1.6×10 6 M −1 s −1 ) and stable coordination at V343C, involving a Cys in each of the three subunits, demonstrates that the internal region of TM2 must move a large distance towards the central axis of the pore during opening. If Cd 2+ coordination is tetrahedral (with water as the fourth ligand) and the bond length of each S-Cd 2+ is ~2.5 Å [38] , [39] , each TM2 would need to move about 10 Å for Cys at V343 to coordinate the metal ion ( Fig. 4e ). Consideration of these constraints, together with the structure of the closed zfP2X4 receptor, leads us to propose a model in which expansion of the gate region of the external pore and constriction of the internal pore are accomplished by straightening the TM2 helix from the steeply angled orientation seen in the zfP2X4 structure towards the normal of the bilayer ( Fig. 6 ). This motion of TM2 could readily explain the Ag + accessibility for one face of TM1 in the open state even without invoking absolute movements of TM1. Moreover, this pore-opening mechanism could explain how stable Cd 2+ bridges involving V343C in all three subunits could form at the central axis in the open state ( Fig. 6 , site a), whereas somewhat weaker bridges involving two Cys residues at S345 in TM2 and a His at position 33 in TM1 could form off the central axis ( Fig. 6 , site b). Although this off-axis bridge involving S345C and H33 would be consistent with a narrowing of the internal pore during opening, the relatively slow rate at which it forms in the presence of ATP (7.7 ± 0.2 × 10 4 M −1 s −1 ) leaves open the possibility that the bridge forms in a more rarely occupied or distorted state. 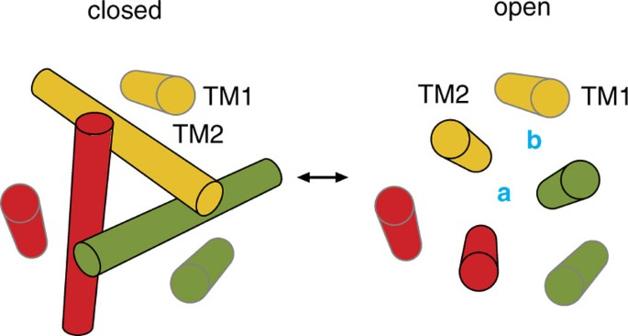Figure 6: Illustrations of the motions of the TM2 helix during opening of P2X receptors. The TM helices are viewed from the extracellular side of the membrane. The coordinating site located at the central axis of the pore is indicated by the letter a, whereas the site located off the central axis is indicated by the letter b. Figure 6: Illustrations of the motions of the TM2 helix during opening of P2X receptors. The TM helices are viewed from the extracellular side of the membrane. The coordinating site located at the central axis of the pore is indicated by the letter a, whereas the site located off the central axis is indicated by the letter b. Full size image One intriguing feature of this model is that it raises the possibility that the internal pore may contain important ion-binding sites involved in determining the ion permeation properties of the channel, in addition to those previously inferred within external regions of the pore [20] , [21] , [22] , [23] , [24] , [29] . All P2X receptors in higher eukaryotes contain an Asp residue (D349 in rP2X2) one helical turn below positions at which we find that Cd 2+ can be stably coordinated at the central axis of the pore, and mutations of this residue either disrupt function [18] , [19] , [40] , [41] or decrease single-channel conductance [29] . In addition, a recent study reported that Cd 2+ could be stably coordinated in the D349C mutant of rP2X2 in the presence of ATP [32] , although the state in which it forms is unclear because the rate of bridge formation is slow (2×10 4 M −1 s −1 ), and the coordinating residues were not defined because stable bridging required a native Cys at position 348 in TM2 and the required number of subunits harbouring the D349C mutation was not tested. It would be interesting to resolve these uncertainties to determine whether D349 is optimally positioned to form a divalent ion-binding site within the inner pore of P2X receptor channels. Perhaps the most interesting feature of the pore-opening model is that it implies that subunit–subunit interactions within the pore domain must undergo substantial rearrangements during opening. The closed state zfP2X4 structure is striking in that subunit–subunit interactions in the pore domain are extremely limited, and can only be seen within the gate region of TM2 between I332 and T339 () [15] . In effect, the gate itself serves to hold the three subunits together. These intersubunit interactions must become further limited as the TM2 helices expand to open the pore, indicating that other subunit–subunit interactions are needed to stabilize the structure of the open pore. Straightening of the TM2 helix would allow TM1 to participate in intersubunit interactions with two adjacent TM2 helices ( Fig. 6 ). Positioning of TM1 at the subunit interface in the open state would be consistent with the off-axis bridge involving an H33 in TM1 and an S345C in two adjacent TM2 helices ( Fig. 5c,d ), and the Ag + accessibility we observed for residues on one face of the TM1 helix in the presence of ATP ( Fig. 2c–e ). Such dramatic restructuring of subunit–subunit interactions within the pore of P2X receptors may help to explain how the ion selectivity of these channels changes when they are continually activated with ATP [42] , [43] , [44] . It will be interesting to explore whether similar pore-opening mechanisms are used in structurally related trimeric cation channels, including acid-sensing ion channels and epithelial sodium channels [17] . Channel constructs Cys mutations were introduced into the rP2X2 receptor channel [45] (generously provided by D. Julius, UCSF) in which Cys9, Cys348 and Cys430 were mutated to Thr (rP2X2-3T) [28] . Concatamers were constructed as previously described [46] , [47] , and confirmed by DNA sequencing as well as western blot. Cell culture and transfection Human embryonic kidney (HEK293) cells were cultured in Dulbecco's modified Eagle's medium supplemented with 10% fetal bovine serum and 10 mg l −1 gentamicin. Trypsin-treated HEK293 cells were seeded onto glass coverslips in six-well plates 1 day before transfection and placed in a 37°C incubator with 95% air and 5% CO 2 . Transfections were performed using FuGENE6 Transfection Reagent. rP2X2 constructs were co-transfected with a green fluorescent protein complementary DNA construct in pGreen-Lantern (Invitrogen) at a ratio of 2:1. Cells were used for whole-cell recording 24–48 h after transfection. Electrophysiology All electrophysiological experiments were conducted in transiently transfected HEK-293 cells with standard whole-cell patch clamp recording. Membrane currents were recorded under voltage clamp at −60 mV using an Axopatch 200B patch clamp amplifier and digitized online using a Digidata 1322A interface board and pCLAMP 9 software. Currents were filtered at 2 kHz using 8-pole Bessel filters, and digitized at 5 or 10 kHz. The standard extracellular solution contained (mM) 140 NaCl, 5.4 KCl, 2 CaCl 2 , 0.5 MgCl 2 , 10 HEPES and 10 D -glucose, adjusted to pH 7.3 with NaOH. The standard pipette solution contained (mM) 140 NaCl, 10 EGTA and 10 HEPES, adjusted to pH 7.0 with NaOH. For the experiments with Ag + , the extracellular solutions contained (mM) 140 NaNO 3 , 5.4 KNO 3 , 10 EDTA and 10 HEPES at pH 7.3, and the intracellular solution contained (in mM) 140 NaCl, 10 EDTA and 10 HEPES at pH 7.0. Stock solutions of MTS reagents, AgNO 3 and CdCl 2 were prepared daily and diluted to the desired concentration in extracellular solution immediately before each experiment. ATP, MTS reagents, Ag + and Cd 2+ were delivered by a rapid perfusion system (BioLogic RSC-200) that effectively changes solutions in 50 ms. Solutions containing ATP were freshly prepared every 2 h. For each Ag + experiment, freshly prepared extracellular solutions containing a total of 1, 10 or 50 μM AgNO 3 were used. The free Ag + concentration in these solutions with 10-mM EDTA was calculated using maxchelator.stanford.edu with appropriate stability constants for our conditions and determined to be 7, 67 and 300 nM, respectively. Ag + has no effect on rP2X2-3T channel currents activated by saturating concentrations of ATP, but produces a reversible enhancement of currents when the channel is activated by EC 50 concentrations of ATP. To examine the accessibility of introduced Cys residues, we used saturating concentrations of ATP and only report modification that is irreversible. Because high concentrations of Ag + (300 nM) evoke significant current in untransfected HEK293 cells, this concentration of Ag + was only used to confirm that a given position is inaccessible to Ag + . Time constants for modification ( τ ) were obtained by fitting relaxations with a single exponential function, and modification rates ( R ) were calculated according to: where [M] is the concentration of thiol-reactive reagent. How to cite this article: Li, M. et al . Pore-opening mechanism in trimeric P2X receptor channels. Nat. Commun. 1:44 doi: 10.1038/ncomms1048 (2010).